Size evolution of highly amphiphilic macromolecular solution assemblies via a distinct bimodal pathway The solution self-assembly of macromolecular amphiphiles offers an efficient, bottom-up strategy for producing well-defined nanocarriers, with applications ranging from drug delivery to nanoreactors. Typically, the generation of uniform nanocarrier architectures is controlled by processing methods that rely on cosolvent mixtures. These preparation strategies hinge on the assumption that macromolecular solution nanostructures are kinetically stable following transfer from an organic/aqueous cosolvent into aqueous solution. Herein we demonstrate that unequivocal step-change shifts in micelle populations occur over several weeks following transfer into a highly selective solvent. The unexpected micelle growth evolves through a distinct bimodal distribution separated by multiple fusion events and critically depends on solution agitation. Notably, these results underscore fundamental similarities between assembly processes in amphiphilic polymer, small molecule and protein systems. Moreover, the non-equilibrium micelle size increase can have a major impact on the assumed stability of solution assemblies, for which performance is dictated by nanocarrier size and structure. Self-assembly schemes provide a simple and tuneable approach for creating a myriad of well-defined nanostructures from designer macromolecules in bulk, thin film and solution environments. Decades of fundamental research provide a foundation for understanding and controlling self-assembled morphologies, making macromolecules pivotal in the development of many emerging nanotechnologies. In particular, polymeric nanostructures in solution have attracted significant attention in the drug delivery, cosmetics, dispersant technology, sensor and nanoreactor arenas [1] , [2] , [3] . Many of the envisioned applications endeavour to exploit solution assemblies as nanocontainers for the encapsulation of small molecule cargoes such as drugs/therapeutics or other reagents, requiring a detailed understanding of the dynamic processes and long-term stability of solution-assembled nanostructures. Amphiphilic macromolecules, such as block copolymers, are promising for the abovementioned applications as molecular design offers enormous chemical versatility and exquisite control over the size and shape of solution assemblies. Like their small molecule surfactant analogues, amphiphilic macromolecules form various nanostructures in aqueous solutions including spherical micelles, cylindrical micelles and vesicle bilayers [4] , [5] , [6] . Of particular interest are the unique material properties conferred by the macromolecular nature of the hydrophobic block, such as extremely low critical aggregation concentrations and exceptionally slow inter-aggregate chain exchange in highly selective solvents such as water [6] , [7] , [8] , [9] . These characteristics overcome key limitations of small molecule aggregates by improving the retention of encapsulated cargoes for drug delivery [6] , [8] and nanoreactor applications [10] . The slow dynamic processes inherent to macromolecular amphiphiles also lead to kinetically trapped structures, requiring careful optimization of preparation conditions to produce well-defined, uniform and reproducible solution assemblies [8] . Many common preparation methods employ cosolvent mixtures to create well-defined and classical solution nanostructures that mirror the morphologies expected from equilibrium thermodynamics (for example, spherical micelles, cylindrical micelles and vesicles) [8] , [11] , [12] . In these cases, the copolymer is dissolved in a common solvent for both polymer blocks, and then a selective solvent is added. This selective solvent normally increases the energy barrier to dynamic processes and potentially allows one to kinetically trap specific morphologies [8] . Several groups have exploited cosolvent processing routes to produce non-equilibrium and exotic nanostructures such as patchy spheres [13] , striped cylinders [13] , [14] and toroids [15] . By manipulating the solvent selectivity for the copolymer constituents, these examples demonstrate the power of cosolvent processing to create complex, hierarchical structures from simple building blocks [8] , [13] . Cosolvent processing principles also are employed regularly in the loading of self-assembled morphologies with various hydrophobic cargoes such as dyes and therapeutic agents for diagnostics and drug delivery applications [16] , [17] , [18] . Cosolvent methods are essential to solubilise both the hydrophobic cargo and amphiphilic copolymer to facilitate efficient encapsulation within self-assembled nanocarriers. As nanocarriers are routinely used in aqueous solution, these preparation methods also hinge on the assumption that the assemblies are kinetically trapped (and nanostructure is preserved) following transfer from an organic/aqueous solution into water. Nanocarrier functionality is directly determined by size and shape, and hence the validity of this assumption is of the utmost importance. However, we note that the resulting metastable nanostructures may rearrange given a sufficiently large driving force [8] . Although the effects of cosolvent introduction on the generation of block copolymer assemblies are well researched [19] , [20] , [21] , [22] , the consequences of cosolvent removal on self-assembled structures typically are overlooked. Although some macromolecular assemblies are known to be kinetically trapped over time scales of days [22] , [23] , [24] or even months [25] , a cohesive understanding of polymeric micelle dynamics is still lacking. This information gap exists because the dynamic processes are influenced by numerous coupled factors that can depend on how far removed the assemblies are from their equilibrium configuration (for example, aggregation number, size and shape) [7] , [9] , [26] , [27] . In general, two mechanisms are considered key for facilitating changes in micelle size and structure: single-chain exchange and micelle fusion/fission ( Fig. 1 ). Near equilibrium, single-chain exchange events dominate the dynamics in both small molecule surfactant and block copolymer micelles [19] , [22] , [28] , [29] , [30] . However, the energetic barrier to chain exchange in macromolecular systems normally is much higher owing to the long-chain hydrophobic block, and this barrier is highly dependent on the solvent selectivity for the polymer blocks [8] , [19] , [23] . Chain exchange events are imperceptibly slow in highly selective solvents [22] , [23] , [25] , yet occur readily in mildly selective solvents [28] , [29] , [30] . 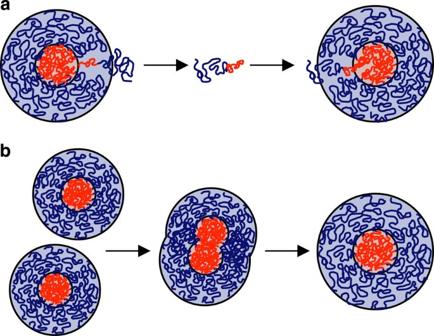Figure 1: Mechanisms for micelle growth. Schematic representation of the common micelle growth mechanisms through (a) single-chain exchange or (b) micelle fusion. In single-chain exchange, a polymer chain escapes from the micelle core, diffuses through solution and then re-inserts into another micelle. In micelle fusion, two micelles collide, the micelle coronas deform and the cores merge to form a larger micelle. Figure 1: Mechanisms for micelle growth. Schematic representation of the common micelle growth mechanisms through ( a ) single-chain exchange or ( b ) micelle fusion. In single-chain exchange, a polymer chain escapes from the micelle core, diffuses through solution and then re-inserts into another micelle. In micelle fusion, two micelles collide, the micelle coronas deform and the cores merge to form a larger micelle. Full size image Meanwhile, far from equilibrium, the dominant dynamic process in macromolecular assemblies is unclear [7] , [9] , [31] , [32] , [33] . Dormidontova [26] used scaling analysis to suggest that micelle fusion is the preferred growth mechanism in this regime, as opposed to the single-chain events that are prevalent near equilibrium. In contrast, other reports argue that the energetic barrier to deform the micelle coronas is too high to permit fusion in these systems, and therefore that only single-chain events are favoured [19] , [34] . Thus, despite the growing importance of understanding dynamics in macromolecular assemblies, the mechanisms governing structural evolution in highly perturbed systems remain unresolved. Herein we show that significant dynamic processes do occur in block copolymer micelles following cosolvent removal, even in highly selective solvents, provided that the system is perturbed sufficiently far from equilibrium. In the absence of agitation, the micelles are stable, consistent with scaling theories that predict insurmountable energy barriers to dynamic processes [19] , [34] . However, gentle agitation, which is not considered in scaling theories, leads to a marked increase in the micelle size. The micelle sizes evolve through a bimodal distribution, in which well-defined step changes in size lead to a monodisperse final nanostructure population with an aggregation number approximately eight times larger than that of the starting population. These results provide the first detailed experimental evidence for a distinct bimodal size distribution of spherical micelles during a fusion-controlled growth process and emphasize the influence of common preparation conditions (for example, cosolvent addition, dialysis, agitation) on the long-term stability of the resulting block copolymer assemblies. Effects of cosolvent removal on micelle size The consequences of cosolvent removal on the dynamics of block copolymer micelles were studied using a poly(butadiene- b -ethylene oxide) or PB-PEO copolymer, with PB and PEO block molecular weights of 3.2 kg mol −1 and 7.9 kg mol −1 , respectively. The low molecular weight and low glass transition temperature of the hydrophobic PB-block permitted investigations into the micelle dynamics independent of entanglement or glassy effects in the micelle core [23] , [25] . Micelles were prepared in water/tetrahydrofuran (THF) cosolvent mixtures using a method analogous to common drug-loading procedures [16] , [17] , [18] . First, the polymer was dissolved in water, resulting in well-defined spherical micelles with PB cores surrounded by PEO coronas. We note that similar micelle sizes were obtained by adding water to dry polymer powder or a thin polymer film, supporting that the micelles in pure water were close to their equilibrium size. After stirring for 72 h, THF was added to the desired cosolvent composition (0–50% by volume THF). Dynamic light scattering (DLS) data showing the temporal changes in micelle solution behaviour following cosolvent removal are provided in Fig. 2 . The initial micelle radii were inversely related to THF content in the cosolvent mixture, as noted by the decrease in hydrodynamic radius versus THF fraction (‹ R h › values at Day −1 in Fig. 2 ) [20] , [21] . The trends noted here were consistent with previous reports showing that adding an organic cosolvent improved the solvent quality for the core block and reduced the core-corona interfacial tension, leading to a reduction in micelle size [20] , [21] . 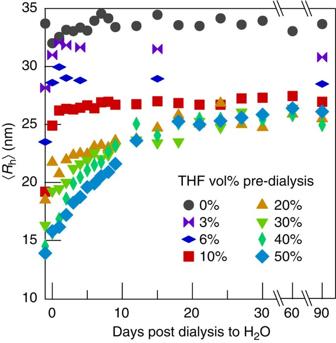Figure 2: DLS study of micelle size evolution. Dynamic light scattering (DLS) data showing average micelle hydrodynamic radii ‹Rh› before (Day −1) and after THF cosolvent removal (Day 0 to Day 90). Day −1 analyses were performed immediately before dialysis against water. Day 0 marks the end of the 24 h transfer of the micelles from the cosolvent into pure water through dialysis. Data were analysed using the second-order cumulant method. The variability in the fitted ‹Rh› value was within 1–3 nm. The polymer concentration was 2 mg ml−1before dialysis into pure water in all cases. Figure 2: DLS study of micelle size evolution. Dynamic light scattering (DLS) data showing average micelle hydrodynamic radii ‹ R h › before (Day −1) and after THF cosolvent removal (Day 0 to Day 90). Day −1 analyses were performed immediately before dialysis against water. Day 0 marks the end of the 24 h transfer of the micelles from the cosolvent into pure water through dialysis. Data were analysed using the second-order cumulant method. The variability in the fitted ‹ R h › value was within 1–3 nm. The polymer concentration was 2 mg ml −1 before dialysis into pure water in all cases. Full size image Following dialysis into pure water (that is, complete THF removal), micelle sizes were unchanged in quiescent solutions, regardless of the initial THF content in the cosolvent mixture ( Supplementary Fig. 1 ). This result was consistent with scaling theories that predict large energy barriers to dynamic processes in macromolecular assemblies [26] , [34] . However, gentle agitation (magnetic stirring at 200 r.p.m., estimated volume average shear rate ~20 s −1 ) [35] led to an unexpected temporal evolution in micelle size that depended on the composition of the cosolvent mixture. The ‹ R h › of micelles prepared in cosolvent mixtures that contained ≤10% by volume THF remained constant over 90 days following THF removal, although these nanostructures were smaller than the micelles prepared in pure water ( Fig. 2 ). This lack of size evolution suggested that those micelles were near equilibrium or unable to overcome the energetic barrier for rearrangement. The stability of micelles prepared from the pure water and low THF content solutions was consistent with reports indicating that PB-PEO micelles should be kinetically trapped in aqueous solutions owing to the highly unfavourable PB-water interaction ( χ PB/water ≈3.5) [23] , [25] . In contrast, micelles prepared in cosolvent mixtures that contained >10% by volume THF exhibited significant size increases in the ≈20 days following THF removal, despite the unfavourable PB-water interaction. The DLS data indicated that the micelles prepared from high THF content mixtures approached a similar final size of ‹ R h ›≈25 nm following transfer into pure water, regardless of their initial size in the cosolvent mixture. Small angle X-ray scattering (SAXS) analyses reinforced the trends seen in the DLS results and provided insight into changes in the micelle size dispersity following cosolvent removal. The shift in primary peak location to higher q -values with increasing THF content ( Fig. 3a ) confirmed the inverse relationship between micelle size and THF content on cosolvent addition. The disappearance of the main peak on Day 3 ( Fig. 3b ) for the specimens made from 30 to 50% by volume THF solutions suggested an appreciable increase in the size dispersity in the days immediately following cosolvent removal. The reappearance of the peak at lower q -values on Day 30 ( Fig. 3c ) indicated that micelles had coalesced into a final population of larger and nearly monodisperse assemblies. The initial increase and subsequent decrease in dispersity suggested the presence of multiple micelle populations during the growth process. Moreover, the final micelle sizes were similar for the specimens made from 10 to 50% by volume THF solutions, supporting the plateau in growth noted in the DLS results. 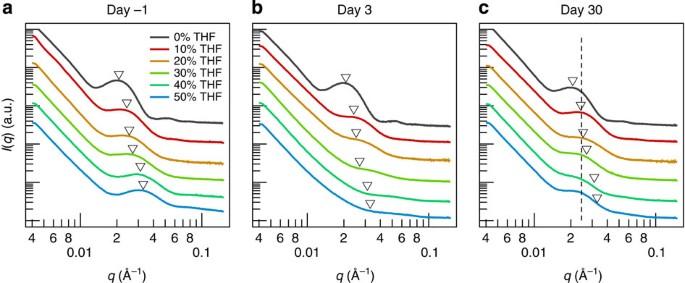Figure 3: SAXS study of micelle size evolution. Small angle X-ray scattering (SAXS) data for micelles prepared in various water/THF mixtures (0–50% by volume THF) on Day −1 before dialysis (a), Day 3 after dialysis (b) and Day 30 after dialysis (c). Triangles mark the peak location before dialysis into pure water. The dashed line highlights the peak location in the samples generated from the⩾10% by volume THF solutions 30 days after dialysis into pure water. SAXS curves were shifted vertically for clarity. Figure 3: SAXS study of micelle size evolution. Small angle X-ray scattering (SAXS) data for micelles prepared in various water/THF mixtures (0–50% by volume THF) on Day −1 before dialysis ( a ), Day 3 after dialysis ( b ) and Day 30 after dialysis ( c ). Triangles mark the peak location before dialysis into pure water. The dashed line highlights the peak location in the samples generated from the ⩾ 10% by volume THF solutions 30 days after dialysis into pure water. SAXS curves were shifted vertically for clarity. Full size image The differences in growth behaviour of the micelles prepared from low versus high THF cosolvent mixtures were reasonable on the basis of the free energy contributions that govern amphiphilic block copolymer self-assembly [20] . The larger micelles formed in the low THF content mixtures likely are close to their equilibrium size and are unable to overcome the energetic barrier to dynamic processes. In contrast, the smaller micelles formed in high THF content mixtures have a larger interfacial area per chain than the micelles formed in pure water, leading to highly unfavourable PB-water interactions following dialysis. A size increase of the smaller micelles reduces the interfacial area per chain and lowers the free energy of the system. Although free energy analyses suggested that the growth of the smaller micelles in water would be energetically favourable, the noted size increase in Figs 2 and 3 was not expected when considering micelle growth mechanisms and their associated energetic barriers in highly amphiphilic systems [19] , [23] , [25] , [26] , [34] , [36] . These results possibly indicated new insights into block copolymer micelle stability and prompted further investigation. Investigation into micelle growth mechanism The growth of PB-PEO micelles following solvent transfer into pure water was examined using small angle neutron scattering (SANS) and cryogenic transmission electron microscopy (cryo-TEM). Specifically, single-chain exchange in water was investigated using SANS by exploiting contrast variations and monitoring the temporal changes in the scattered intensity ( Fig. 4a ) [22] , [28] , [29] , [30] , [37] . Initially, separate PB-PEO and PB- d PEO (poly(butadiene- b -ethylene oxide- d 4 )) micelle solutions were prepared in an H 2 O/D 2 O mixture. These separate solutions were mixed at time t =0, giving rise to a maximum in scattered intensity owing to contrast between the coronas and solvent ( I(q ) values at t =0 in Fig. 4b ). After mixing the separate PB-PEO and PB- d PEO micelle solutions, two possible outcomes were considered. In the first scenario, chain exchange would occur, leading to randomization of the PB-PEO and PB- d PEO chains in the micelles. This mixing of the chains would reduce the corona/solvent contrast and decrease the scattered intensity, as the isotopic composition of the solvent was selected to contrast-match a randomly mixed PEO/ d PEO corona (lower scattered intensity I(q ) values for pre-mixed PEO/ d PEO corona sample in Fig. 4b ). In the second scenario, single-chain exchange would not occur and the scattered intensity would remain nearly constant with time. 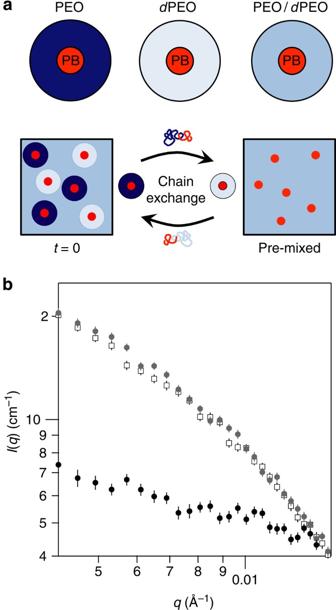Figure 4: SANS results showing negligible chain exchange over 10 days. (a) Illustration of small angle neutron scattering (SANS) experiments used to probe chain exchange in micelle solutions. The scattering of initially segregated poly(butadiene-b-ethylene oxide) (PB-PEO, top left) and poly(butadiene-b-ethylene oxide-d4) (PB-dPEO, top centre) micelles was monitored in solvents that were contrast-matched to the corona in a mixed micelle system (PB-PEO/dPEO, top right). (b) SANS curves showing the measured scattered intensity from pre-mixed PB-PEO/PB-dPEO micelles (black circles) and mixtures of PB-PEO and PB-dPEO micelles immediately after mixing (open squares) or 10 days after mixing (grey circles) in D2O/H2O at 25 °C. Figure 4: SANS results showing negligible chain exchange over 10 days. ( a ) Illustration of small angle neutron scattering (SANS) experiments used to probe chain exchange in micelle solutions. The scattering of initially segregated poly(butadiene- b -ethylene oxide) (PB-PEO, top left) and poly(butadiene- b -ethylene oxide- d 4 ) (PB- d PEO, top centre) micelles was monitored in solvents that were contrast-matched to the corona in a mixed micelle system (PB-PEO/dPEO, top right). ( b ) SANS curves showing the measured scattered intensity from pre-mixed PB-PEO/PB- d PEO micelles (black circles) and mixtures of PB-PEO and PB- d PEO micelles immediately after mixing (open squares) or 10 days after mixing (grey circles) in D 2 O/H 2 O at 25 °C. Full size image For our system, the scattered intensity did not decrease over 10 days ( Fig. 4b ), supporting the second scenario and a lack of appreciable chain exchange by micelle fusion/fission and/or single-chain events. This lack of exchange found in our work is consistent with previous reports on the non-ergodicity of PB-PEO micelles in aqueous solutions and the highly unfavourable PB-water interaction [23] , [25] , [38] . Moreover, recent reports have demonstrated that the energy barrier to single-chain exchange only depends on the properties of the hydrophobic block and not on the micelle size/aggregation number [19] , [28] , [39] . Thus, the results in Fig. 4 support that single-chain exchange is highly unfavourable in our system and therefore not contributing to the micelle growth noted in Figs 2 and 3 . As chain exchange was not prevalent in this PB-PEO system, fusion processes were examined as the other mechanism that could promote micelle reorganization. To visualize the micelle growth, cryo-TEM was employed to follow the temporal evolution of a micelle solution (10 mg ml −1 in 43% by volume THF) over a 21-day period following cosolvent removal. The resulting micrographs are shown in Fig. 5a , in which the darker domains correspond to the dense PB cores, whereas the fainter halos correspond to the PEO coronas [40] , [41] . Note that the hexagonal packing in the Day 10, 16 and 21 samples was an artefact of sample preparation ( Supplementary Fig. 2 ). The core sizes were extracted from the images, and the corresponding frequency histograms are shown in Fig. 5b . The core radii at Day 0 were described by a single and nearly monodisperse distribution centred at 5–6 nm. Surprisingly, a second distinct distribution of core radii centred at 10–11 nm appeared after 1 day. This second distribution corresponded to an approximate eightfold increase in core volume or aggregation number from the initial distribution, in which the small and large micelle populations contained aggregation numbers of approximately 100 and 800, respectively ( Supplementary Fig. 3 ). The distinct bimodal distribution persisted throughout 10 days, with the population weighting shifting from the smaller to larger distribution over time. By Day 16 to Day 21, the core size distribution exhibited a single and nearly monodisperse population at 10–11 nm, consistent with the time scales determined from DLS ( Fig. 2 ). Similar behaviour was found for the samples prepared from 30% by volume and 50% by volume THF solutions ( Supplementary Fig. 4 and Supplementary Discussion ), suggesting that all specimens prepared at high THF contents grew through a fusion-controlled process. 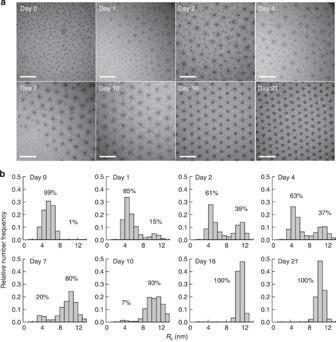Figure 5: Cryo-TEM studies of micelle size evolution. (a) Cryogenic transmission electron microscopy (cryo-TEM) images showing changes in micelle core radii (Rc) over 21 days post-dialysis. The polymer concentration was initially 10 mg ml−1, and the THF content was 43% by volume before dialysis. Scale bar, 100 nm. (b) Corresponding histograms of micelle sizes obtained from analysis of cryo-TEM images. The relative percentages of the smaller (Rc<8 nm) and larger (Rc⩾8 nm) core radii populations are shown on the histograms. Sample sizes for each histogram ranged between 450 and 3,000 micelles. Figure 5: Cryo-TEM studies of micelle size evolution. ( a ) Cryogenic transmission electron microscopy (cryo-TEM) images showing changes in micelle core radii (R c ) over 21 days post-dialysis. The polymer concentration was initially 10 mg ml −1 , and the THF content was 43% by volume before dialysis. Scale bar, 100 nm. ( b ) Corresponding histograms of micelle sizes obtained from analysis of cryo-TEM images. The relative percentages of the smaller (R c <8 nm) and larger (R c ⩾ 8 nm) core radii populations are shown on the histograms. Sample sizes for each histogram ranged between 450 and 3,000 micelles. Full size image Concentration dependence of size evolution Fusion events are predicted to follow second-order kinetics and should increase in rate as the micelle concentration increases [27] , [42] . Therefore, the size evolution was examined as a function of micelle concentration using DLS ( Supplementary Fig. 5 ), cryo-TEM ( Fig. 6a,b ) and SANS ( Fig. 6c,d ). DLS data could be fit with either a monomodal or bimodal distribution ( Supplementary Fig. 6 ) and consequently could not distinguish concentration-dependent size changes ( Supplementary Fig. 7 ). This significant uncertainty in determining the concentration dependence with DLS necessitated more sensitive cryo-TEM and SANS studies. The cryo-TEM images show that on Day 10/11, the 2 mg ml −1 and 5 mg ml −1 solutions still contained an appreciable bimodal population of micelles, whereas the 10 mg ml −1 solution had transitioned to primarily larger micelles ( Fig. 6b ). These micrographs suggested that the relative weighting of the larger population increased with micelle concentration and further supported that the micelles grew through fusion. 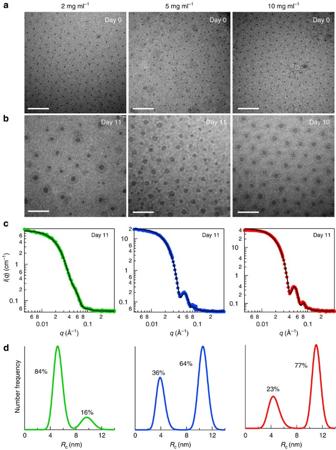Figure 6: Effects of solution concentration on micelle size evolution. Cryogenic transmission electron microscopy (cryo-TEM) micrographs showing changes in micelle core radii between Day 0 (a) and Day 10 or Day 11 (b) for several polymer concentrations. The initial polymer concentrations were 2 mg ml−1, 5 mg ml−1and 10 mg ml−1. After dialysis, the concentrations followed the same trend but were approximately half of the initial concentrations. In each case, the THF content was 43% by volume before dialysis into water. Scale bar, 100 nm. (c) Small angle neutron scattering (SANS) data (points) and fits (solid lines) for micelle solutions at different concentrations. (d) Corresponding number frequency distribution of core radii from fits to SANS data. Samples for the SANS experiments were prepared in 43% by volume THF and dialyzed against D2O, and SANS experiments were performed at Day 11 post-dialysis to D2O. The relative percentages of the smaller (Rc<8 nm) and larger (Rc⩾8 nm) core radii populations are shown on the frequency curves. The sensitivity of the number frequencies from the SANS data modelling was approximately ±5% for the 2 mg ml−1data and ±15% for the 5 mg ml−1and 10 mg ml−1data. Figure 6: Effects of solution concentration on micelle size evolution. Cryogenic transmission electron microscopy (cryo-TEM) micrographs showing changes in micelle core radii between Day 0 ( a ) and Day 10 or Day 11 ( b ) for several polymer concentrations. The initial polymer concentrations were 2 mg ml −1 , 5 mg ml −1 and 10 mg ml −1 . After dialysis, the concentrations followed the same trend but were approximately half of the initial concentrations. In each case, the THF content was 43% by volume before dialysis into water. Scale bar, 100 nm. ( c ) Small angle neutron scattering (SANS) data (points) and fits (solid lines) for micelle solutions at different concentrations. ( d ) Corresponding number frequency distribution of core radii from fits to SANS data. Samples for the SANS experiments were prepared in 43% by volume THF and dialyzed against D 2 O, and SANS experiments were performed at Day 11 post-dialysis to D 2 O. The relative percentages of the smaller (R c <8 nm) and larger (R c ⩾ 8 nm) core radii populations are shown on the frequency curves. The sensitivity of the number frequencies from the SANS data modelling was approximately ±5% for the 2 mg ml −1 data and ±15% for the 5 mg ml −1 and 10 mg ml −1 data. Full size image Although microscopy provides unique structural insights (for example, an unexpected bimodal distribution) that were difficult to identify solely through scattering analysis [43] , [44] , typical TEM sample sizes are small (~10 3 micelles) compared with the much larger sample size (~10 15 micelles) that is examined with scattering techniques. Thus, SANS experiments were performed to ensure that the measured micelle size distributions were not influenced by cryo-TEM sample preparation. In these experiments, the micelle coronas were contrast-matched to the solvent (D 2 O) by blending PB-PEO and PB- d PEO polymers, thereby probing only the PB core size distribution. The SANS data showed a marked difference in micelle populations for the 2 mg ml −1 sample versus the higher concentration samples ( Fig. 6c ). The distinct maxima and minima in the 5 and 10 mg ml −1 data indicated that a significant population of larger micelles were present in the higher concentration samples. Also, the maxima and minima were located at approximately the same q -values, supporting that the larger micelles were the same size in both samples. These trends were substantiated by modelling the data using a bimodal distribution of Schulz spheres, which resulted in significantly better fits than the model for monomodal spheres ( Supplementary Fig. 8 and Supplementary Discussion ). The resulting bimodal fits to the SANS data ( Fig. 6c ) and corresponding number frequency distributions of core radii ( Fig. 6d ) are presented for the different polymer concentrations. The bimodal core distribution centred at R c ≈5 nm and ≈10 nm was in good agreement with the cryo-TEM results. In addition, the SANS results indicated that the relative weighting of the larger to smaller core population increased with increasing polymer concentration, again supporting the fusion mechanism for micelle growth. The bimodal micelle growth behaviour in our PB-PEO micelle solutions has critical implications for block copolymer micelle stability in highly selective solvents. Specifically, we show that when micelle assemblies are perturbed far enough from their equilibrium size, the micelles can evolve through a fusion-controlled process, and moreover, through a distinct bimodal distribution that is separated by multiple fusion events ( Fig. 7 ). 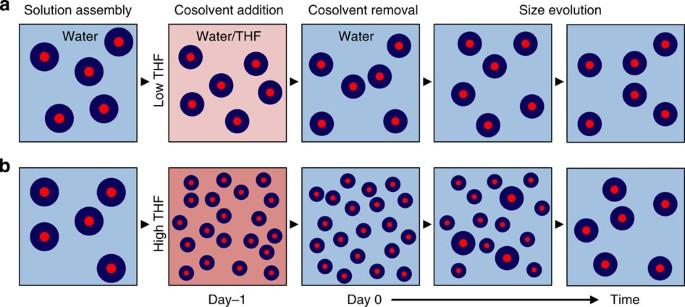Figure 7: Summary of micelle size evolution. Schematic representation of changes in micelle size after cosolvent addition and removal. (a) Poly(butadiene-b-ethylene oxide) (PB-PEO) micelles self-assemble in pure water, decrease in size following THF cosolvent addition (<10% by volume) and remain kinetically trapped after solvent transfer to pure water. Micelles prepared in solutions containing low THF contents are not perturbed far from their equilibrium size and therefore do not undergo significant size relaxation. (b) Increasing the THF content (for example, 40% by volume) and subsequently removing the cosolvent perturbs the micelles far from their equilibrium size in water, leading to size relaxation through a bimodal pathway. Figure 7: Summary of micelle size evolution. Schematic representation of changes in micelle size after cosolvent addition and removal. ( a ) Poly(butadiene- b -ethylene oxide) (PB-PEO) micelles self-assemble in pure water, decrease in size following THF cosolvent addition (<10% by volume) and remain kinetically trapped after solvent transfer to pure water. Micelles prepared in solutions containing low THF contents are not perturbed far from their equilibrium size and therefore do not undergo significant size relaxation. ( b ) Increasing the THF content (for example, 40% by volume) and subsequently removing the cosolvent perturbs the micelles far from their equilibrium size in water, leading to size relaxation through a bimodal pathway. Full size image The energy barrier to micelle fusion is related to the corona chain stretching and is expected to scale with aggregation number [26] , [45] , [46] . Accordingly, the energy barrier should rise with increasing aggregation number, and the fusion of intermediate sized micelles should be slower than the fusion of smaller micelles. Based on this scaling, we would expect to see distinct intermediate populations if the micelles were growing by stepwise two-body collisions. Theoretical [26] and computational work [42] posited that distinct multimodal size distributions would exist for micelles undergoing stepwise fusion growth. This behaviour differs from that of micelles growing through single-chain events, which would be characterized by a shifting monomodal size distribution [42] , [47] , [48] . However, the distinct bimodal distribution found here does not reflect either of these predictions and instead suggests an alternate growth mechanism. Bimodal distributions often are indicative of a nucleation and growth mechanism (that is, cooperative self-assembly). Cooperative self-assembly processes have been reported in numerous systems including proteins [49] , peptide-based molecules [50] , small molecules [49] , [51] and nanoparticles [52] and are characterized by a bimodal distribution of small oligomers and larger aggregates. In our system, the small micelles may fuse to form metastable intermediates, which then rapidly fuse with additional smaller micelles to produce a bimodal size distribution. This proposed growth mechanism is potentially similar to the cooperative micellization processes in small molecule amphiphiles, in which the final micelle size is imposed by repulsive interactions between the head groups [53] . Similarly, corona chain repulsion may limit the micelle growth seen here, leading to the final size plateau independent of the initial size. Notably, this final size was smaller than micelles formed by directly dispersing the polymer in water ( Fig. 2 ), underscoring the path-dependent and kinetically controlled self-assembly in macromolecular systems. Interestingly, the micelle size evolution critically depended on solution agitation, suggesting that the growth may be a shear-induced and/or interfacial phenomenon. Agitation has been shown to influence the formation of macromolecular assemblies [54] , [55] , [56] and is known to significantly affect protein stability [35] , [57] , [58] , [59] . In particular, several reports indicate that proteins can aggregate during agitation by adsorbing to and subsequently unfolding at the air/water interface [57] , [58] , [59] . Amphiphilic block copolymers also are known to assemble at air/water interfaces [60] , [61] , which may imply that the bimodal growth pathway is owing to an interface-induced micelle nucleation and growth process. Clearly, further quantitative studies are needed to distinguish the detailed mechanism and associated kinetics to fully understand the potential shear and/or interfacial effects on the long-term stability of macromolecular assemblies. In summary, our findings highlight the considerable influence of cosolvent preparation methods on the long-term stability of macromolecular assemblies and demonstrate the strong interplay between thermodynamic versus kinetic constraints in these systems. We show that micelle fusion/fission events occur in amphiphilic block copolymer micelles when the system is perturbed far from equilibrium, even in highly selective solvents. Notably, the unexpected micelle growth was likely an interfacial and/or shear phenomenon, leading to a bimodal size distribution separated by multiple fusion events with no dominant intermediate populations. Although the effects of perturbation and agitation often are overlooked in polymeric assemblies, our results accentuate similarities between the processing effects in polymeric systems and those that are influential in small molecule and protein assemblies. This intimate relationship between processing conditions and subsequent dynamics has critical implications on the stability of macromolecular-based nanocarriers. Furthermore, these results emphasize the need for more quantitative investigations into the underlying mechanisms affecting micelle stability to enable a thorough understanding of the complex dynamic processes in amphiphilic block copolymer solution assemblies. Polymer synthesis PB-PEO and PB- d PEO were synthesized by anionic polymerization using established protocols [21] , [62] . The molecular weight of the PB precursor ( M n =3.2 kg mol −1 , Ð =1.06, 1, 2-PB content=92±1%) was determined using matrix-assisted laser desorption/ionization time-of-flight mass spectrometry and proton nuclear magnetic resonance ( 1 H NMR) spectroscopy. The dispersity was determined from size exclusion chromatography with polystyrene standards. The PB-PEO ( M n =11.1 kg mol −1 , w PEO =0.71, Ð =1.08) and PB- d PEO ( M n =11.0 kg mol −1 , w d PEO =0.71, Ð =1.09) polymers were characterized using size exclusion chromatography and 1 H NMR. The molecular weights of PB-PEO and PB- d PEO were determined using the molecular weight of the PB-OH precursor from matrix-assisted laser desorption/ionization time-of-flight mass spectrometry and the polymer composition from 1 H NMR. Micelle solution preparation Micelle solutions were prepared by adding 18 MΩ water to dry polymer powder and stirring the solutions for 3 days. Then, THF (Optima, 99.9%, Fisher Scientific) was added to achieve the desired cosolvent composition, and the solutions were stirred for an additional 3 days. The micelle solutions were dialyzed (Spectra/Por Regenerated Cellulose Dialysis Tubing, MWCO=12–14 kg mol −1 ) against water for 24 h with three water changes to completely remove the cosolvent. Day 0 refers to the end of the dialysis. Solutions were magnetically stirred (200 r.p.m.) at room temperature between experiments. The polymer concentration post-dialysis was determined at the end of the studies by either measuring the ultraviolet–visible absorbance of the polymer solution samples or by drying a known volume of the solution specimen and weighing the remaining polymer. For the ultraviolet–visible experiments, the absorbances obtained from the solution samples were compared with a calibration curve for micelle solutions with known concentrations. The samples used to generate the calibration curves were made from known mass concentrations of either PB-PEO dissolved in 18 MΩ water or 88% by mass PB- d PEO/12% by mass PB-PEO dissolved in D 2 O ( Supplementary Fig. 9 ). Micelle solutions employed for the calibration studies were stirred for at least 3 days before measuring the ultraviolet–visible absorbance. The absorbance of the dialyzed solutions was measured using a Thermo Scientific Nanodrop ND-1000 ultraviolet–visible spectrophotometer at least 20 days after dialysis. As expected, owing to expansion of the dialysis tubing as a result of osmotic pressure, the calculated sample concentrations following dialysis were approximately half the initial concentrations. DLS DLS experiments were performed using a Brookhaven Instruments Light Scattering System (BI-200SM, Brookhaven Instruments Corporation) equipped with a Lexel Laser operating at 488 nm. Measurements were made at a scattering angle of 90°, and all experiments were performed at 25 °C. The autocorrelation functions were fit with the quadratic cumulant expansion [63] . Additional analyses are given in Supplementary Figs 6 and 7 and the Supplementary Discussion . Literature values for the viscosity and refractive index of water/THF mixtures used to analyse the DLS data before cosolvent removal are listed in Supplementary Table 1 [64] . SAXS SAXS experiments were performed on the 12-ID-C beamline at the Advanced Photon Source (APS) at Argonne National Lab. Data were collected using an incident X-ray wavelength ( λ ) of 0.73 Å and a sample-to-detector distance of 5.3 m to give a scattering wave vector range from 0.004 Å −1 < q <0.15 Å −1 . The scattering wave vector is defined as q =(4 π / λ ) sin ( θ /2); θ is the scattering angle. Cryo-TEM Samples for cryo-TEM were prepared using an FEI Vitrobot at 22 °C and relative humidity of 100%. Before sample loading, carbon-coated copper TEM grids (Quantifoil R 2/1 or Quantifoil S 7/2) were plasma etched for 60 s. A 3 μl drop of micelle solution was pipetted onto the grid inside the sample chamber. Using an automated system, the grid was blotted with filter paper twice to remove the excess solution. Blot offset (none), blot time (3 s), wait time (1 s) and drain time (1 s) were consistent for each sample. After blotting, grids were submerged in liquid ethane to vitrify the sample. Grids were stored in liquid nitrogen before imaging. Imaging was performed on a Tecnai G2 12 Twin TEM operating at 120 kV. Images were recorded using a Gatan CCD camera at a nominal underfocus to enhance phase contrast. The temperature of the sample probe was maintained between −176 and −180 °C during imaging. PB core radii were determined using ImageJ software [65] . First, the image noise was suppressed using a despeckle algorithm, and a bandpass filter was applied. Subsequently, a contrast threshold was used to remove the background, leaving the outlined area of PB cores ( Supplementary Fig. 10 ). The core radii were calculated from the core areas, assuming that the PB cores were spherical and that their 2D projections were circular. Multiple images (6–12) were analysed from different grid locations, with a total sample size between 450 and 3,000 micelles per histogram. Bin sizes for the histograms were 1 nm. SANS Samples for chain exchange experiments were prepared as follows. Pre-mixed PB-PEO/PB- d PEO (50% by mass PB-PEO) micelle solutions were prepared using the following approach. First, the PB-PEO and PB- d PEO polymers were blended in benzene, stirred overnight, then freeze-dried to ensure complete solvent removal. Then, the polymer blend was dissolved in a D 2 O/H 2 O mixture (64% by volume D 2 O) at a concentration of 2 mg ml −1 polymer in solvent and stirred for 3 days. The isotopic composition of 64% by volume D 2 O was chosen to contrast-match a perfectly mixed PEO/ d PEO corona. Individual PB-PEO and PB- d PEO micelle solutions for post-mixed experiments were prepared by dissolving each dry polymer powder in a separate D 2 O/H 2 O mixture (64% by volume D 2 O) and then stirring for 3 days. Both solutions had a final concentration of 2 mg ml −1 polymer in solvent. For t =0 sample, equal volumes of the PB-PEO and PB- d PEO solutions were mixed and analysed with SANS. For the t =10 days sample, equal volume of the PB-PEO and PB- d PEO solutions were mixed, magnetically stirred (200 r.p.m.) at room temperature for 10 days, and analysed with SANS. Samples to determine the micelle core size distribution using SANS were prepared using blended PB-PEO/PB- d PEO (12% by mass PB-PEO) polymers to contrast-match the micelle corona to the D 2 O solvent. The PB-PEO and PB- d PEO were blended in benzene, stirred overnight and freeze-dried. Micelle solutions of the blended polymers were prepared in water/THF cosolvent mixtures as described above and dialyzed against deuterium oxide (D 2 O, 99.9% D, Cambridge Isotopes). After dialysis, the solutions were magnetically stirred (200 r.p.m.) at room temperature. SANS experiments were performed on the NG-7 30 m SANS instrument at the National Institute of Standards and Technology, Center for Neutron Research. An incident wavelength of 6.0 Å was used with sample-to-detector distances of 1, 4 and 13.5 m to cover a q -range from 0.004 Å −1 < q <0.4 Å −1 . All measurements were performed at ambient temperature. The data were reduced and analysed in the IGOR Pro software package (WaveMetrics) using the standard procedures provided by NIST [66] . Additional SANS experiments were performed on the CG-2 General Purpose SANS instrument at the High Flux Isotope Reactor at Oak Ridge National Laboratory (ORNL). A sample-to-detector distance of 14 m was used with an incident neutron wavelength ( λ ) of 4.75 Å to cover a scattering vector ( q ) range from 0.006 Å −1 < q <0.09 Å −1 . Scattering data were recorded for 5 min, and all experiments were performed at 25 °C. SANS data were reduced using the procedures provided by ORNL. The data were corrected for background scattering, empty cell scattering, sample transmission, sample thickness and detector sensitivity and were normalized to an absolute scale using a pre-calibrated secondary standard. How to cite this article: Kelley, E. G. et al. Size evolution of highly amphiphilic macromolecular solution assemblies via a distinct bimodal pathway. Nat. Commun. 5:3599 doi: 10.1038/ncomms4599 (2014).